Control of the spin geometric phase in semiconductor quantum rings Since the formulation of the geometric phase by Berry, its relevance has been demonstrated in a large variety of physical systems. However, a geometric phase of the most fundamental spin-1/2 system, the electron spin, has not been observed directly and controlled independently from dynamical phases. Here we report experimental evidence on the manipulation of an electron spin through a purely geometric effect in an InGaAs-based quantum ring with Rashba spin-orbit coupling. By applying an in-plane magnetic field, a phase shift of the Aharonov–Casher interference pattern towards the small spin-orbit-coupling regions is observed. A perturbation theory for a one-dimensional Rashba ring under small in-plane fields reveals that the phase shift originates exclusively from the modulation of a pure geometric-phase component of the electron spin beyond the adiabatic limit, independently from dynamical phases. The phase shift is well reproduced by implementing two independent approaches, that is, perturbation theory and non-perturbative transport simulations. Geometric phases arise in wave systems [1] where the parameters of the wave function are cycled around a circuit. Such phase factors can be observed via interference of waves traversing different paths. Berry [1] has shown that the electron spin wave function in an adiabatic evolution acquires a geometric phase that depends only on the geometry of the traversed path in the parameter space. As a consequence, the geometric phase is robust against dephasing. This is in contrast to the time-dependent dynamical phase of a particle [2] , [3] , [4] . Experimentally, geometric-phase factors have been observed in various systems [5] , [6] . However, the geometric phase of an electronic spin has never been directly observed and manipulated independently of the dynamical phase before. Here we demonstrate the control of the geometric phase of an electron spin in a mesoscopic semiconductor device in which an array of rings forms interference paths. The experiment shows geometric phases beyond the adiabatic limit [7] . A geometric-phase shift of the Aharonov–Casher (AC) effect [8] , [9] , [10] is induced with an in-plane magnetic field and measured in an interference pattern of the electron current. Our findings show manipulation of the geometric phase independently of the dynamical phase without introducing additional geometric-phase factors such as the Aharonov–Bohm phase. Concept of present experiment Spins in a magnetic field acquire a dynamical phase, which physically corresponds to phase accumulation because of the spin precession around the magnetic field. In a mesoscopic ring system with an inhomogeneous magnetic field, the spins acquire also a geometric phase that depends on the path of the spin. As an example, consider a one-dimensional (1D) ring in a textured magnetic field [11] as shown in Fig. 1a . The magnetic field seen by a propagating electron along the ring subtends, from its rest frame, a solid angle in the magnetic-field space. The spin acquires not only a dynamical phase but also a geometric phase, which is proportional to the solid angle ( Fig. 1b ). 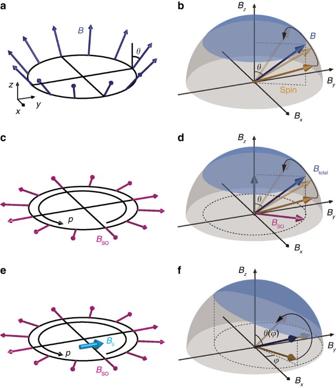Figure 1: Schematic illustration of spin geometric phases in quantum rings. (a) Quantum ring of radiusrplaced in a crown-like magnetic field with an angleθwith respect to thezaxis. (b) In the electron’s rest frame, the textured field subtends a solid angle (blue) in a round trip around the ring. In adiabatic transport, the solid angle is proportional to the geometric phase. Spin precession aroundBis associated with the dynamical phase. (c) Rashba SO coupling induces an effective in-plane magnetic fieldBSOperpendicular to the electron momentumP. (d) In non-adiabatic transport, the effective magnetic field has an additionalzcomponent proportional toω0pr/2. The geometric phase is proportional to the solid angle subtended by the total effective magnetic field. (e) The geometric phase in a Rashba ring can be controlled by adding an in-plane field. (f) The in-plane field modulates the geometric phase via changing the solid angle subtended by the total effective field. Figure 1: Schematic illustration of spin geometric phases in quantum rings. ( a ) Quantum ring of radius r placed in a crown-like magnetic field with an angle θ with respect to the z axis. ( b ) In the electron’s rest frame, the textured field subtends a solid angle (blue) in a round trip around the ring. In adiabatic transport, the solid angle is proportional to the geometric phase. Spin precession around B is associated with the dynamical phase. ( c ) Rashba SO coupling induces an effective in-plane magnetic field B SO perpendicular to the electron momentum P . ( d ) In non-adiabatic transport, the effective magnetic field has an additional z component proportional to ω 0 pr /2. The geometric phase is proportional to the solid angle subtended by the total effective magnetic field. ( e ) The geometric phase in a Rashba ring can be controlled by adding an in-plane field . ( f ) The in-plane field modulates the geometric phase via changing the solid angle subtended by the total effective field. Full size image The Bychkov–Rashba spin-orbit (SO) coupling [12] can be used to create an effective in-plane magnetic-field texture ( Fig. 1c ). The coupling is induced at an interface between semiconductor layers having different energy gaps by an electric field perpendicular to the layers (say along the z axis). It is a relativistic effect where an electron travelling through an electric field feels an effective SO magnetic field B SO , the direction of which is perpendicular both to the electric field and a wave vector k , that is, B SO ∝ α R ( k × e z ). Here the electric field enters through the Rashba SO-coupling constant α R that is therefore electrically tunable with a top-gate electrode [13] , [14] , and e z denotes a unit vector in z direction. This effective Rashba field couples to the electron spin, which acquires dynamical and geometric phases in the transport around the ring [15] , [16] , [17] . Interference of these spin-related phases gives rise to conductance oscillations when α R is varied [18] , [19] , [20] . Recently, the SO-induced geometric phase has been extracted [21] from a detailed analysis of spin-interference effects as a function of the SO-coupling constant α R and the ring radius r . In a 1D Rashba ring placed in the x – y plane, a travelling electron has a non-zero wave vector k only in the in-plane direction because of the electrostatic confinement along e z . Consequently, the effective field B SO seen by the electron always points in the radial direction (see Fig. 1c ). However, if the revolution frequency ω 0 around the ring is comparable to the spin-precession frequency ω SO , spin transport is non-adiabatic. As a result the electron spin does not exactly precess around B SO (see refs 22 , 23 ); spin eigenstates are no longer parallel to B SO and the corresponding polar angle, θ , satisfies , with being the effective mass of an electron and ħ the reduced Planck’s constant, as if there was an effective magnetic field normal to the ring’s plane besides B SO as depicted in Fig. 1d . This is in analogy to NMR experiment where an rf magnetic field yields a static out-of-plane field in a rotating frame of reference. Hence, an electron spin in the Rashba ring acquires a geometric phase, which corresponds to the solid angle subtended by the spin eigenstates. Now, consider a Rashba ring with an external magnetic field applied parallel to the ring plane as shown in Fig. 1e : the total magnetic field seen by the electron is uniformly tilted towards the applied field direction, which changes the solid angle in the magnetic-field space ( Fig. 1f ). As we will show, this allows for controlled modulation of the pure geometric phase independently of the dynamical phase. We emphasize that the separation of the geometric and dynamical phases has not been achieved in mesoscopic spin systems so far: the SO-coupling constant α R and the ring radius r modulate both the geometric and dynamical phases simultaneously through the degree of adiabaticity, Q R . In-plane field dependence of the AC effect In our experiment, an array of 40 × 40 rings ( Fig. 2a ) and a Hall bar have been fabricated lithographically from a shallow InGaAs quantum well (see ref. 24 for the basic properties). The Hall bar and the ring array are in the same current path and they have been covered with the same top-gate electrode. The electrical resistance has been measured with a standard ac lock-in technique at a temperature of 1.5 K with a liquid helium cryostat where we can apply magnetic fields both perpendicular and parallel to the ring plane. 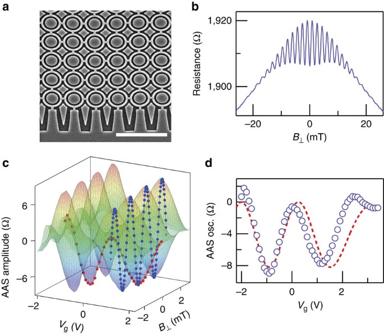Figure 2: Altshuler–Aronov–Spivak and AC oscillations in an InGaAs-based ring array. (a) Scanning electron microscope image of an array of 40 × 40 InGaAs-based rings. The radius of each ring is 0.6 μm. Scale bar, 5 μm. (b) Magnetoresistance of the ring array in perpendicular magnetic fieldsB⊥at 1.5 K shows the AAS oscillations. The gate voltageVg=1.1 V. (c)Vgdependence of the AAS oscillations amplitude. (d)Vgdependence of the AAS amplitude atB⊥=0, corresponding to the AC effect in the TR paths. The red dashed line represents the theoretical prediction of equation (2). To plot the dashed line, we used the relation between the Rashba SO-coupling constantαRversusVg, which was obtained from the Shubnikov–de Haas analysis13in the Hall bar. Figure 2b shows the Altshuler–Aronov–Spivak (AAS) effect in the ring array at a gate voltage of 1.1V as a function of the perpendicular magnetic-field strength. Figure 2: Altshuler–Aronov–Spivak and AC oscillations in an InGaAs-based ring array. ( a ) Scanning electron microscope image of an array of 40 × 40 InGaAs-based rings. The radius of each ring is 0.6 μm. Scale bar, 5 μm. ( b ) Magnetoresistance of the ring array in perpendicular magnetic fields B ⊥ at 1.5 K shows the AAS oscillations. The gate voltage V g =1.1 V. ( c ) V g dependence of the AAS oscillations amplitude. ( d ) V g dependence of the AAS amplitude at B ⊥ =0, corresponding to the AC effect in the TR paths. The red dashed line represents the theoretical prediction of equation (2). To plot the dashed line, we used the relation between the Rashba SO-coupling constant α R versus V g , which was obtained from the Shubnikov–de Haas analysis [13] in the Hall bar. Full size image We study the control of the spin geometric phase via the AC effect [8] , [9] , [10] , the electromagnetic dual of the Aharonov–Bohm effect. Specifically, in our system, the AC effect is realized as the gate modulation of spin interference. The AAS amplitude oscillates with the gate voltage, as shown in Fig. 2c , indicating the gate modulation of the spin phase. This oscillatory behaviour of the magnetoresistance at zero (perpendicular) external field is visualized in Fig. 2d . Because of disorder in the samples and the ensemble average over the ring array, pairs of time-reversed (TR) paths, that is, the path pairs travelling in opposite directions around the ring, contribute predominantly to the interference pattern in the magnetoresistance. The AC effect in the TR paths gives rise to the resistance modulation given by [25] , [23] where δ R α R ≠ 0 and δ R α R = 0 are, respectively, the electrical resistance with and without Rashba SO coupling in a ring. Equation (2), plotted as the red dashed line in Fig. 2d , is in agreement with experiment. The phase of the cosine function in equation (2) shows that the AC phase comprises two components, namely, a dynamical component 2 πQ R sin θ and a geometric one −2 π (1−cos θ ). The latter exactly represents the solid angle subtended by the spin eigenstates in the Rashba ring ( Fig. 1d ). The dependence of the AC effect on the in-plane magnetic field in experiment is shown in Fig. 3a,b . In Fig. 3a , the gate voltage is translated to the Rashba SO-coupling constant α R by using the relation obtained from the Shubnikov–de Haas analysis [13] in the Hall bar. As is applied, the amplitude of the AC effect is suppressed because of spin-induced TR symmetry breaking [26] (see the Supplementary Note 1 ). Further, the AC oscillations exhibit a quadratic shift with towards positive gate voltages, that is, weaker Rashba SO-coupling strengths. In the following, we explain the observed shift by the sole modulation of the geometric phase as shown in Fig. 1f . 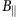Figure 3:Geometric-phase shift because of an in-plane magnetic field. In the upper panels (a,c,e), the AC oscillations are shown as a function of the Rashba SO-coupling constantαRand the in-planefield. In the lower panels (b,d,f), the AC oscillations are shown for four differentas a function of the gate voltage,Vg. (a,b)-field dependence of the AC effect (experiment). The AC oscillations shift to weaker SO fields with increasing, which is an indication of a geometric-phase shift. Notations P1-P4 indicate peaks and dips of the AC oscillations. The dashed lines inaare guides for the eye. The dashed lines inbrepresent the zero-line of the AAS amplitude. (c,d) Perturbation theory for a 1D Rashba ring with a smallfield. The chain line represents rough estimation of the validity of the perturbation expansion. Inc, a suppression factor26of the AC oscillation amplitude is applied in addition to the phase shift described by the equation (3). The dashed lines indshow the zero-line of the cosine function in the equation (3). (e,f) Numerical calculations of the AC effect in disordered multimode rings. The six transverse modes per spin are considered and the electron mean free path is 2 μm. In all calculations, the g-factor. The dashed lines infshow the baseline, which corresponds to the resistance atαR=0. Because of the weak antilocalization effect, the AAS oscillations have a negative amplitude against this line and depend onVg. Figure 3: Geometric-phase shift because of an in-plane magnetic field . In the upper panels ( a , c , e ), the AC oscillations are shown as a function of the Rashba SO-coupling constant α R and the in-plane field. In the lower panels ( b , d , f ), the AC oscillations are shown for four different as a function of the gate voltage, V g . ( a , b ) -field dependence of the AC effect (experiment). The AC oscillations shift to weaker SO fields with increasing , which is an indication of a geometric-phase shift. Notations P1-P4 indicate peaks and dips of the AC oscillations. The dashed lines in a are guides for the eye. The dashed lines in b represent the zero-line of the AAS amplitude. ( c , d ) Perturbation theory for a 1D Rashba ring with a small field. The chain line represents rough estimation of the validity of the perturbation expansion. In c , a suppression factor [26] of the AC oscillation amplitude is applied in addition to the phase shift described by the equation (3). The dashed lines in d show the zero-line of the cosine function in the equation (3). ( e , f ) Numerical calculations of the AC effect in disordered multimode rings. The six transverse modes per spin are considered and the electron mean free path is 2 μm. In all calculations, the g-factor . The dashed lines in f show the baseline, which corresponds to the resistance at α R =0. Because of the weak antilocalization effect, the AAS oscillations have a negative amplitude against this line and depend on V g . Full size image Perturbation theory and numerical transport calculations To evaluate the effect of in-plane magnetic fields on the geometric phases in the limit of small , we employ perturbation theory for a 1D Rashba ring (see the Methods section). The phase shift is calculated to first order in . We find that the AC interference between TR pairs of paths leads to conductance oscillations where and . Further, k F is the Fermi wave number, is the Landé g -factor and μ B is the Bohr magneton. By comparing equations (1) and (3), we find that provides an additional phase 2 π φ quadratic in . As plotted in Fig. 3c,d , equation (3) reproduces the observed phase shift within the energy range of small Zeeman energy (due to ) compared with the kinetic and Rashba SO-coupling energies. A similar quadratic shift in the interference peak positions has been recently calculated also for weakly coupled rings [27] . To determine the origin of the AC-phase shift, we calculate a geometric-phase contribution φ AA using eigenstates calculated to first order in the in-plane field: with ϕ being the azimuthal angle in the ring plane and j being an integer. By comparing equations (1, 2, 3) and (6), we confirm that the perturbation term φ has a purely geometric origin, at least to first order in the in-plane field strength. This is because electron spins in the TR interference paths experience a uniaxial field, which does not yield a dynamical phase difference through the spin precession. Hence, our central result is that the observed shift of the AC phase is induced by the modulation of the pure geometric phase of an electron spin. Note that the wave number enters into the denominator of the geometric-phase shift term φ , equation (4). In our samples the conducting channel contains at least six transverse modes, each having a unique wave number. To take into account the effect of the multiple transport modes and for an adequate treatment of field strengths beyond the perturbative limit, we employ the numerical recursive Green’s function method [28] (see the Supplementary Note 2 ). Results calculated at fixed carrier density 1.0 × 10 16 m −2 are shown in Fig. 3e,f . The geometric shift of the AC oscillations occurs even in the presence of multiple modes (see the Supplementary Note 3 ). 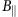Figure 4:Geometrical shift of peak and dip positions of the AC oscillations with an in-plane field. The vertical axis represents the quantity of the AC-phase shift in units of Rashba SO-coupling constant, ΔαR. Notations P1-P4 are the peak and dip positions of the AC phase (seeFig. 3). The results are shown for experiment (filled symbols), perturbation theory (solid lines) and numerical analysis (open symbols). The chain and dashed lines are eye guides for the experimental and numerical results, respectively. A hysteresis of the gate voltage is subtracted from the experimentally observed shift inFig. 3a. The plots are shifted vertically for adjusting the peaks/dips at. Figure 4 shows the comparison of the geometric shift in experiment (filled symbols) with the perturbation theory (solid lines) and the non-perturbative numerical calculations (open symbols) at peak and dip positions of the AC oscillations (P1–P4; see Fig. 3 ). The carrier density in the numerical calculations is increased with gate voltage (see the Supplementary Note 2 ). The perturbation theory for a single transverse mode is in good agreement with experiment in the regime of strong SO coupling (P1 and P2). This indicates that the phase shift is dominated only by a few modes or just the lowest one, presumably because of stronger decoherence for higher transverse modes, which have the smaller wave numbers along the ring. The discrepancy is significant at weak SO-coupling regions (P3 and P4) that are beyond the limit of validity of the perturbation expansion. We note that wave numbers associated with the modes in multimode numerical calculations depend on the energy level spacing in the confining channel of the ring. Numerical calculations assume a square-shaped potential, which may lead to the overestimation of the phase shift at P1. Further, in the numerical model a transition from weak antilocalization to weak localization with changing Rashba SO coupling results in the increased background resistance at small SO fields (see Fig. 3f ). As a result, the positions of P3 and P4 may shift. However, almost all the results show the peaks and dips shift towards weak Rashba SO coupling, that is, positive gate voltages. We are thus able to reasonably simulate and explain the experimentally observed spin-phase shift by both numerical calculations and the perturbation theory. Figure 4: Geometrical shift of peak and dip positions of the AC oscillations with an in-plane field . The vertical axis represents the quantity of the AC-phase shift in units of Rashba SO-coupling constant, Δ α R . Notations P1-P4 are the peak and dip positions of the AC phase (see Fig. 3 ). The results are shown for experiment (filled symbols), perturbation theory (solid lines) and numerical analysis (open symbols). The chain and dashed lines are eye guides for the experimental and numerical results, respectively. A hysteresis of the gate voltage is subtracted from the experimentally observed shift in Fig. 3a . The plots are shifted vertically for adjusting the peaks/dips at . Full size image For further evidence, we have measured the radius dependence of the -induced phase shift. 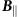Figure 5:Radius dependence of the geometrical phase shift with an in-plane field. The vertical axis represents the phase shift of the AC oscillations in units of radians (one period of the AC oscillations corresponds to 2πrad). Experimental results are plotted as the open (filled) symbols forr=0.6 μm (1.1 μm) sample. The lines are the perturbation theory, withr=0.6 μm (dashed) andr=1.1 μm (solid). The notations P1-P4 represent the peak and dip positions of the AC phase (seeFig. 3). Figure 5 shows the comparison of the shift in samples of rings with r =0.6 and 1.1 μm. We see that both in experiment and in the perturbation theory, geometric-phase shift increases with the ring radius. This confirms an important prediction of our theory contained in the equations (3) and (4). From the comparison between experiment and the theory, the diamagnetic shift of energy is negligible in our samples because the diamagnetic effect should not have the radius dependence. To the best of our knowledge, this is the first experimental demonstration of the pure geometric-phase control of an electron spin in solid-state devices. We conclude that this multiparameter control of the spin geometric phase may pave the way for future spintronic applications, such as geometric-gate operation [29] of a solid-state flying qubit or control of persistent spin currents in a mesoscopic ring [11] , [30] , which may have potential applications for non-volatile memory devices. Figure 5: Radius dependence of the geometrical phase shift with an in-plane field . The vertical axis represents the phase shift of the AC oscillations in units of radians (one period of the AC oscillations corresponds to 2 π rad). Experimental results are plotted as the open (filled) symbols for r =0.6 μm (1.1 μm) sample. The lines are the perturbation theory, with r =0.6 μm (dashed) and r =1.1 μm (solid). The notations P1-P4 represent the peak and dip positions of the AC phase (see Fig. 3 ). Full size image Sample fabrication and measurements The sample was epitaxially grown on a (001) InP substrate by metal organic chemical vapour deposition. It consists of, from the bottom, In 0.52 Al 0.48 As (200 nm, buffer layer)/In 0.52 Al 0.48 As (6 nm, carrier supply layer; Si-doping concentration of 4 × 10 18 m −3 )/In 0.52 Al 0.48 As (15 nm, spacer layer)/In 0.53 Ga 0.47 As (2.5 nm, quantum well)/In 0.70 Ga 0.30 As (10 nm, quantum well)/In 0.53 Ga 0.47 As (2.5 nm, quantum well)/InP (5 nm, stopper layer)/In 0.52 Al 0.48 As (20 nm, barrier layer)/AlAs (1.5 nm, barrier layer)/In 0.52 Al 0.48 As (5 nm, cap layer). An array of 40 × 40 rings and a Hall bar (70 × 280 μm 2 ) have been fabricated by means of e-beam lithography and reactive-ion etching. To form an ohmic contact, AuGeNi was used (annealing temperature of 275 °C, 7 min). As a top-gate insulator, a 200-nm-thick Al 2 O 3 layer was deposited by atomic layer deposition. A Cr/Au top-gate electrode was fabricated on the insulator layer. A four-terminal standard lock-in technique has been used to measure the perpendicular magnetoresistance of the ring array as a function of the gate voltage and the in-plane magnetic field. At a given gate voltage, the Rashba SO-coupling constant and the carrier density in the ring structure can be estimated by measuring the Shubnikov–de Haas oscillations in the Hall bar. Perturbation theory We introduce a perturbative approach for studying the effect of small in-plane magnetic fields in the conductance of 1D rings subject to Rashba SO coupling. We demonstrate that the in-plane field acts on the geometrical spin phase alone without contributing to dynamical phases at the lowest perturbative order, allowing the controlled manipulation of geometrical phases. The Hamiltonian reads with Here H 0 is the unperturbed Hamiltonian of a 1D Rashba ring of radius r lying in the x – y plane parametrized by the azimuthal angle ϕ . We have defined ω 0 =ħ/ mr 2 and ω SO =2 α R /ħ r as the characteristic frequencies of the kinetic and SO Rashba terms, respectively, together with the polar Pauli matrices σ r =cos ϕ σ x +sin ϕ σ y and σ ϕ =−sin ϕ σ x +cos ϕ σ y . The third term in equation (8) guarantees H 0 to be Hermitian [22] , losing relevance for large momenta. The Δ H in equation (9) is a perturbation on H 0 by an in-plane magnetic field along the x direction, with the corresponding Larmor frequency. The unperturbed eigenstates | n , λ , s › 0 of H 0 (with spin s =↑,↓, travel sense λ =±1, and orbital wave numbers n ≥0) are [23] where θ is the inclination of the local spin-quantization axis with respect to the z axis given by tan θ = ω SO / ω 0 ≡ Q R . Notice that θ does not depend on any quantum number, being shared by all eigenstates. The corresponding eigenenergies are Where ↑ spins are defined to maximize the eigenenergies. We notice that states with opposite travel sense | n ,−, s › 0 and | n −1,+, s › 0 are degenerated (that is, ). In addition, we find that , namely, the perturbation Δ H does not mix degenerate states. This means that we can apply a non-degenerate perturbation theory. We further notice that an additional degeneracy ( ) arises in the unperturbed system for vanishing Rashba coupling ( Q R =0), meaning that the perturbative approach we present here is not valid for . We calculate the perturbed eigenstates | n , λ , s › and eigenenergies to the lowest order in ω B . Taking into account that 0 ‹ n ±1, λ , s |Δ H | n , λ , s › 0 = λs (ħω B /4)sin θ and 0 ‹ n ±1, λ , − s |Δ H | n , λ , s › 0 =ħ ω B (cos θ ± s )/4, we find (by following, for example, the textbook by Sakurai [31] ) with normalization constant , and We calculate the ring conductance by following the procedure introduced in (refs 23 , 25 ). This is based on the 1D Landauer formula , where the conductance G is determined by the quantum probabilities of transmission T σσ′ =| t σσ′ | 2 (with amplitudes t σσ′ ) for incoming (outgoing) spins σ′ (σ). We consider strongly coupled contacts at diametrically opposed locations ϕ =0 and ϕ = π . Because of the energy splitting, incoming spin carriers with Fermi energy E F entering at ϕ =0 can propagate coherently through the ring along four possible channels with (non-integer) wave numbers depending on spin ( s ) and travel sense ( λ ). The are determined by solving in equation (16) and the relative weight of each propagation channel is given by the projection of the incoming spin state on the corresponding spin eigenstates, equation (15), at the entrance point. We assume that, because of strong coupling to the contacts, the carriers propagate directly from the entrance ( ϕ =0) to the exit ( ϕ = π ) point along the shortest paths without any additional winding (see Fig. 6a ). 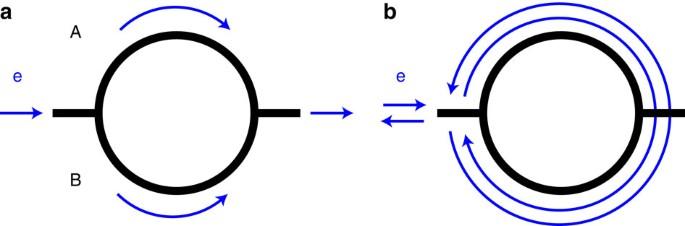Figure 6: Leading paths contributing to coherent spin transport in mesoscopic rings. (a) Interference of paths A and B leads to the AC conductance oscillations in ballistic systems. (b) TR paths lead to the AAS conductance oscillations in disordered multimode systems. After interference, we find by summing over all spin indices, with Figure 6: Leading paths contributing to coherent spin transport in mesoscopic rings. ( a ) Interference of paths A and B leads to the AC conductance oscillations in ballistic systems. ( b ) TR paths lead to the AAS conductance oscillations in disordered multimode systems. Full size image where we assumed a large electron density corresponding to in equations (15) and (16), in agreement with the experimental conditions. The conductance then reads The result of equation (20) holds for single ballistic rings. For an ensemble of rings subject to shape fluctuations and/or disorder, instead, the main contribution to the sample-averaged conductance comes from TR paths leading to the AAS oscillations (see Fig. 6b ). By following a similar procedure (taking into account that TR paths contribute to the transmission probability T through the reflection probability R by unitarity T + R =1), we find an AAS conductance which applies to the reported experiment. The φ of equation (19) corresponds to a phase shift in the AC conductance introduced by the in-plane magnetic field. It is quadratic in the field’s strength ω B and proportional to . The latter illustrates the known fact that spin dynamics under Zeeman coupling depends on the electrons velocity [32] , in contrast to Rashba coupling. We further notice that φ is an increasing function of the ring’s radius r . To demonstrate the geometric nature of φ, we first notice in equations (20) and (21) that , where and are the unperturbed contributions to the dynamical and geometrical phases, correspondingly, with Ω 0 the solid angle described by the unperturbed spin eigenstates over the ring (see ref. 23 ). The limit of adiabatic spin dynamics, where purely geometrical Berry phases arise [1] , corresponds to Q R →∞(θ→ π /2). For a finite Q R (0<θ< π /2), the spin dynamics is non-adiabatic and the geometrical phase (depending explicitly on Q R ) is referred to as the Aharonov–Anandan phase [7] . For the perturbed eigenstates, by defining , the geometric-phase contribution φ AA can be extracted as There we find that the magnetic shift φ is purely geometric. This means that, at the lowest order of perturbation, the in-plane magnetic field modifies the eigenstate spin texture without contributing to the dynamical spin phase. More explicitly, from equation (24) we find ΔΩ=−2 π φ showing that the in-plane field perturbs the spin eigenstates by reducing the solid angle with respect to the unperturbed case. This means that the perturbation hinders adiabatic spin dynamics: In the regime (with unperturbed spinors along θ → π /2) spins are lifted from the ring’s plane by the in-plane magnetic field. The full Aharonov–Anandan geometric phase in the perturbed system reads (mod 2 π ) γ=− π [(1−cos θ )− ϕ ] for single ballistic rings ( Fig. 6a ) and γ =−2 π [(1−cos θ )− ϕ ] for rings ensembles in AAS configuration ( Fig. 6b ). How to cite this article: Nagasawa, F. et al . Control of the spin geometric phase in a semiconductor quantum ring. Nat. Commun. 4:2526 doi: 10.1038/ncomms3526 (2013).